High-pressure radiative conductivity of dense silicate glasses with potential implications for dark magmas The possible presence of dense magmas at Earth’s core–mantle boundary is expected to substantially affect the dynamics and thermal evolution of Earth’s interior. However, the thermal transport properties of silicate melts under relevant high-pressure conditions are poorly understood. Here we report in situ high-pressure optical absorption and synchrotron Mössbauer spectroscopic measurements of iron-enriched dense silicate glasses, as laboratory analogues for dense magmas, up to pressures of 85 GPa. Our results reveal a significant increase in absorption coefficients, by almost one order of magnitude with increasing pressure to ~50 GPa, most likely owing to gradual changes in electronic structure. This suggests that the radiative thermal conductivity of dense silicate melts may decrease with pressure and so may be significantly smaller than previously expected under core–mantle boundary conditions. Such dark magmas heterogeneously distributed in the lower mantle would result in significant lateral heterogeneity of heat flux through the core–mantle boundary. The current structure of Earth’s interior is believed to have developed through dynamic differentiation from a global magma ocean in the early Earth [1] , [2] , [3] , [4] , [5] . Elucidation of the heat-transport properties of silicate melts in the deep Earth is fundamental to understanding the evolution and structure of Earth’s interior. The possible presence of dense, gravitationally stable silicate melts at the bottom of the current mantle, as a remnant of a deep magma ocean, has been proposed to explain observations of anomalously low seismic velocities above the core–mantle boundary (CMB) [6] , [7] , [8] , [9] . Thus, heat flux through the CMB region would strongly depend on the thermal conductivity, both lattice-vibrational ( k lat ) and radiative ( k rad ), of such dense silicate melts, as well as that of constituent minerals of the lower mantle [10] . However, the thermal properties of such silicate melts under relevant high-pressure conditions are poorly understood, while there have been several experimental studies on the thermal conductivity of lower mantle minerals such as magnesium-rich silicate perovskite (bridgmanite) and ferropericlase [11] , [12] , [13] , [14] , [15] . Direct measurements of thermal conductivity on silicate melts under ultrahigh-pressure conditions remain a great challenge and are currently beyond experimental capabilities. Alternatively, silicate glasses have been studied as analogues for quenched silicate melts to simulate high-pressure melt behaviour [16] , [17] , [18] , [19] , [20] , [21] . Recent experimental research on the possible spin-pairing electronic transition of iron in silicate glasses at mid-lower mantle pressures [22] has renewed interest in understanding the thermal transport mechanisms in dense silicate melts at the bottom of the mantle, as changes in the optical properties of iron-bearing phases associated with spin transitions may significantly influence the radiative component of thermal conductivity. In this work, we conducted visible and near-infrared optical absorption and synchrotron Mössbauer spectroscopic measurements of iron-enriched silicate glasses at high pressures up to 85 GPa to clarify the potential influences of pressure-induced electronic structure changes in dense silicate melts on the radiative part of the thermal conductivity. Our results suggest that radiative thermal conductivities of iron-enriched dense silicate melts may become significantly smaller with increasing pressure, compared with those of the constituent minerals of the lower mantle. Optical absorption measurements Optical absorption spectra are associated with energy levels corresponding to different electronic configurations of each 3 d transition metal ion in various coordination sites, and the characteristics of absorption bands in visible to near-infrared spectra reflect energy separations between electronic configurations differing in symmetry in non-cubic coordination environments [23] . Knowledge of the pressure dependence of optical absorption bands of iron-bearing dense silicate glasses is therefore essential to understand changes in high-pressure electronic configurations of the glasses and thereby to infer the radiative part of the thermal conductivity. 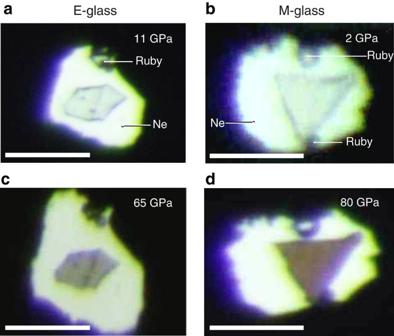Figure 1: Optical images of the glass samples under pressure in the DAC. (a) E-glass at 11 GPa and 300 K; (b) E-glass at 65 GPa and 300 K; (c) M-glass at 2 GPa and 300 K; and (d) M-glass at 80 GPa and 300 K. Pressure medium is neon and the white scale bar is 100 μm long. Two types of silicate glasses were used as analogues for dense silicate melts at the CMB: one with (Mg 0.8 Fe 0.2 )SiO 3 composition (E-glass) to isolate the effect of iron [22] , and the other with a multicomponent basaltic composition (M-glass) ( Table 1 ) to simulate a more realistic compositional system at the CMB [6] , [9] , [24] , [25] . In the optical absorption measurements, both samples visibly became optically darker with pressure, as shown in Fig. 1 . The pressure evolution of the measured absorption spectra is shown in Fig. 2 . We observed significant increases in absorption coefficients with increasing pressure by up to a factor of 3 for E-glass and by an order of magnitude for M-glass, particularly in the visible region above wavenumbers of ~10,000 cm −1 . At low pressures (<20 GPa), E-glass has a broad absorption maximum ~13,000 cm −1 . At higher pressures, we observed new broad peaks at ~15,000 and ~20,000 cm −1 . Peaks in absorption spectra for the multicomponent M-glass are not as clearly evident as those determined for E-glass throughout the range of pressures in this study. Table 1 Chemical composition of basaltic composition multicomponent silicate glass. Full size table Figure 1: Optical images of the glass samples under pressure in the DAC. ( a ) E-glass at 11 GPa and 300 K; ( b ) E-glass at 65 GPa and 300 K; ( c ) M-glass at 2 GPa and 300 K; and ( d ) M-glass at 80 GPa and 300 K. Pressure medium is neon and the white scale bar is 100 μm long. 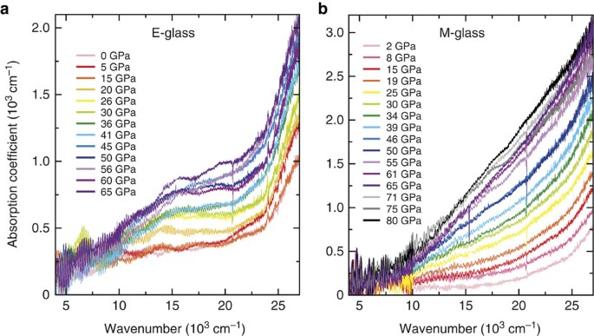Figure 2: Optical absorption spectra of glass samples under pressure at room temperature. (a) E-glass and (b) M-glass. The absorption coefficient was calculated usingα=Aln10/d, whereA=log10(I0/I);I0andIare the reference and sample signals, respectively; anddis the sample thickness measured using white light interferometry at ambient pressure and calculated at high pressure using an isothermal equation of state43,44. Full size image Figure 2: Optical absorption spectra of glass samples under pressure at room temperature. ( a ) E-glass and ( b ) M-glass. The absorption coefficient was calculated using α = A ln10/ d , where A =log 10 ( I 0 / I ); I 0 and I are the reference and sample signals, respectively; and d is the sample thickness measured using white light interferometry at ambient pressure and calculated at high pressure using an isothermal equation of state [43] , [44] . Full size image Synchrotron Mössbauer spectroscopic measurements In situ high-pressure synchrotron Mössbauer spectroscopic measurements in the energy domain were performed on E-glass using the BL11XU beamline of SPring-8, Japan [26] . As shown in Fig. 3a , statistically sufficient Mössbauer spectra were obtained using measurement times between 3 and 6 h. Hyperfine structure parameters were also determined by distribution analysis of the Mössbauer spectra ( Fig. 3b,c ). Above 20 GPa, we observed a new quadrupole doublet (sites 1 and 2), derived from a low isomer shift (IS; ~0.67 mm s −1 relative to α-Fe) and moderate quadrupole splitting (QS; ~1.6 mm s −1 ). If the nearest neighbour atoms around iron are oxygen, in principle, the IS should increase with an increase in the Fe–O coordination number. However, as shown in Fig. 3b , the IS derived from the new quadrupole doublet shows the opposite trend to that expected for pressure-induced coordination number changes. Alternatively, this trend can be interpreted as a change in the electronic state in the absence of significant changes in coordination number, which may relate to the formation of Fe 2+ with a different electronic configuration from that expected at lower pressures. Given that the IS for Fe 2+ with low spin states in common compounds is around −0.3–0.4 mm s −1 , our IS data, exhibiting intermediate values between high and low spin, indicate the appearance of Fe 2+ with an intermediate spin state, rather than a complete transition to low spin states. This intermediate spin state should have fewer unpaired electrons than the high spin state, which would explain the relatively small value of QS (1.5 mm s −1 ; Fig. 3c ). Recent high-pressure synchrotron X-ray Raman scattering analysis of MgSiO 3 glass suggests that pressure-induced topological changes occur below ~20 GPa (ref. 17 ). Such a drastic topological change, including both bond length and bond angle, may also be one possible explanation for the appearance of the new quadrupole doublet, given that the IS normally has an extremely low value (~0.7 mm s −1 ) if a planar coordination geometry, such as (FeO 4 ) 6− , is formed in the local structure [27] . The formation of the planar coordination geometry can also explain the relatively low QS values (~1.5 mm s −1 ) at ~20 GPa (refs 28 , 29 ). Although a recent X-ray emission spectroscopic study of iron-bearing silicate glass showed a precipitous change in spin state of iron at ~75 GPa (ref. 22 ), no clear evidence for such a discontinuous feature was observed in the present study, which may require reconsideration of the previously proposed iron partitioning behaviour in silicate melt under pressure [22] . Very recent experimental work on high-pressure Mössbauer spectra of Mg-, Fe- and Al-bearing silicate glass has also shown the absence of such a precipitous change in spin state with pressure [30] . 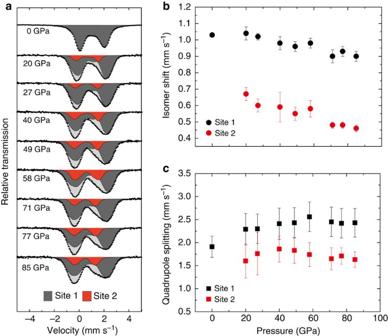Figure 3: Mössbauer transmission spectra and hyperfine structure parameters. Mössbauer transmission spectra determined for E-glass between 0 and 85 GPa (a) and hyperfine structure parameters (b,c). (b) Isomer shift (IS) and (c) quadrupole splitting (QS). Above 20 GPa, a new quadrupole doublet (sites 1 and 2) was observed, derived from a low IS and moderate QS. Error bars are ±1σfrom the mean value. Figure 3: Mössbauer transmission spectra and hyperfine structure parameters. Mössbauer transmission spectra determined for E-glass between 0 and 85 GPa ( a ) and hyperfine structure parameters ( b , c ). ( b ) Isomer shift (IS) and ( c ) quadrupole splitting (QS). Above 20 GPa, a new quadrupole doublet (sites 1 and 2) was observed, derived from a low IS and moderate QS. Error bars are ±1 σ from the mean value. Full size image The present study on iron-enriched silicate glasses indicates a drastic increase in absorption coefficients with increasing pressure, which is possibly owing to changes in electronic structure around the iron atoms. If applicable also to silicate melts in the deep Earth, such changes would affect their radiative thermal conductivity, as the radiative thermal conductivity is based on the emission of electromagnetic waves generated by the thermal motion of charged electrons, which is strongly correlated with the electronic structure of the material. Changes in the intensities of absorption bands with pressure are governed by probabilities of electronic transitions between the split 3 d orbital energy levels, which depend on the spin state or the number of unpaired electrons in a transition metal ion, the location of cation in a coordination site and interactions with next-nearest-neighbour cations [23] . On the other hand, the QS occurs owing to interaction of the nuclear quadrupole moment with the gradient of the electric field that arises from the asymmetry of the field by all the charges surrounding the nucleus. This is highly analogous to the splitting of 3 d orbitals that occurs in transition metals such as iron as a result of crystal field splitting. Therefore, the optical absorption data are closely related to the QS [31] , which gives us information on the radiative thermal conductivity behind the changes in the electronic configurations. Although the effect of temperature requires further exploration to obtain better insight into melts, recent high-pressure radiative thermal conductivity measurements on Earth’s deep minerals [11] , [32] and previous Mössbauer measurements on glasses/liquids [33] , [34] show that the effect of temperature on the optical properties of minerals and on the electronic configurations of glasses/liquids is fairly moderate, which suggests that the analogy in electronic configurations between glass and melt works well. Very recently, Sanloup et al . [35] reported structural changes in molten basalt up to pressures of 60 GPa by means of in situ synchrotron X-ray diffraction, and they have successfully shown that changes in the Si–O coordination number of molten basalt are highly consistent with those observed in silica glass [36] , [37] , [38] , thereby providing experimental evidence in support of the validity of the analogy between silicate glasses and melts in atomic structure. The present data obtained from silicate glasses with representative compositions for dense silicate melt [6] , [9] , [24] , [25] thus indicate the possible effect of pressure-induced changes in electronic configurations, including the spin states of iron, on the thermal properties of melts. Under such assumptions, the radiative component of thermal conductivity, k rad ( T ) was calculated as follows: where n is the refractive index, α is the measured absorption coefficient, I (ν, T ) is the Planck function and T is the temperature. Initial refractive indices of 1.55 and 1.57 were adopted for E-glass and M-glass, respectively [39] , [40] , and a slight pressure dependence of the refractive indices of both silicate glasses was assumed based on compilations from previous literature [41] . Although thermal conditions at the bottom of the mantle are poorly constrained, temperatures are expected to be >3,000 K. We have therefore calculated the radiative contribution to thermal conductivity of the silicate melts up to 7,000 K ( Fig. 4 ), using our experimental absorption spectra. As shown in Fig. 4 , the radiative conductivity increases with temperature and decreases with pressure for both components. Under the highest pressure conditions, the radiative thermal conductivities approach 3.2 and 2.8 W m −1 K −1 at 7,000 K for E-glass and M-glass, respectively. The radiative thermal conductivity of materials with constant absorbance has been believed to be proportional to the third power of temperature (that is, T 3 ). However, the temperature dependence of radiative thermal conductivity estimated in the present study is significantly lower than that expected for a T 3 relationship. The radiative conductivities for both components increase only by a factor of 8–9 from 2,000 to 7,000 K, which is ~5 times more slowly than expected if a T 3 dependency is assumed. This weak temperature dependence may be derived from the non-flat shape of the absorption spectra, indicating an increase in absorption at higher energies. 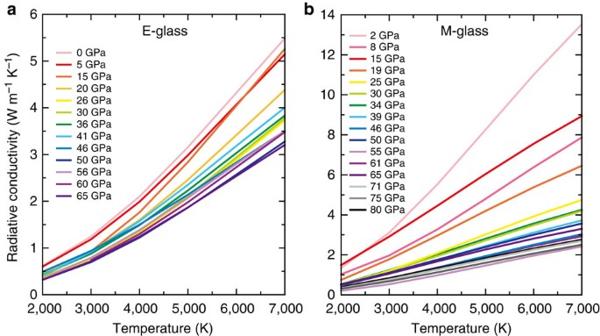Figure 4: Estimated radiative thermal conductivity. Estimated radiative thermal conductivity of E-glass (a) and M-glass (b) as a function of temperature to 7,000 K. The radiative thermal conductivity was calculated using equation (1). Figure 4: Estimated radiative thermal conductivity. Estimated radiative thermal conductivity of E-glass ( a ) and M-glass ( b ) as a function of temperature to 7,000 K. The radiative thermal conductivity was calculated using equation (1). Full size image A significantly smaller contribution to heat transfer by radiative conductivity in silicate melt strongly affects heat flow at the CMB. The possible presence of dense, gravitationally stable magmas at the base of the mantle may represent remnants of a basal magma ocean that was present in the early Earth, which in turn may explain the presence of ultralow seismic velocity zones (ULVZs) above the CMB [6] , [7] , [8] . The results presented here suggest that the radiative thermal conductivity of basaltic melt, calculated from the results of M-glass, under lowermost mantle conditions (at ~130 GPa and ~3,000 K) is estimated to be ~0.19 m −1 K −1 . Although experimental data on the radiative thermal conductivity for silicate perovskite, the principal mineral phase in the lower mantle, under lowermost mantle conditions are still inconclusive [11] , [13] , we find that dense silicate melts with basaltic composition are ~5–25 times less radiatively conductive than the silicate perovskite phase with representative lower mantle iron contents under conditions at the base of the mantle. This remarkable contrast at high pressures indicates the formation of deep magmas with higher heat absorption than the surrounding solid mantle phases. Such dense and dark magmas at the CMB could also act as a trap for heat from the underlying outer core. Seismological mapping at the CMB by detailed waveform modelling studies showed that ULVZs exist as laterally distributed thin layers over a wide region [8] , [42] . The distribution of ULVZs correlates strongly with flux-weighted hot spot locations, which have been interpreted to represent a large-scale lower mantle thermal upwelling referred to as a ‘superplume’ [8] , [42] . A heterogeneous distribution of such dense magmas with low radiative thermal conductivity would result in lateral heterogeneity of heat flux through the CMB, thus potentially constraining the locations of stable hot mantle plumes rooted in the CMB. This conclusion is based on the assumption that the lattice thermal conductivity does not somehow compensate for the reduced radiative conductivity of the deep magma. As there are no experimental data for silicate melts under high pressure, we can only conjecture that the liquids normally have smaller lattice thermal conductivity than the solids owing to decrease in the phonon mean free path. Thus, the lattice component is expected to enhance, rather than mitigate, the effects described here. Direct measurement of thermal properties for silicate melts will ultimately lead to a better understanding of this issue, and substantial efforts are still required to estimate the lattice contribution to thermal conductivity of silicate melt at relevant pressures and temperatures. Sample preparation We synthesized two iron-enriched silicate glasses with representative compositions in MgO–FeO–SiO 2 and multicomponent systems as analogues for dense silicate melts at the CMB. Fe-enriched enstatite glass (E-glass) with a chemical composition of (Mg 0.8 Fe 0.2 )SiO 3 was prepared by mixing stoichiometric amounts of SiO 2 , MgO and Fe 2 O 3 (95% enriched with 57 Fe). The mixture of oxides was placed in a platinum crucible and melted under reducing conditions using a H 2 /CO 2 gas-flow furnace at 1,300 °C and subsequently quenched by immersing the base of the crucible in water. A transmission 57 Fe Mössbauer spectrum of the starting material, E-glass, was collected to determine the valence state of iron using a triangular velocity constant acceleration Mössbauer spectrometer with a nominal 50 mCi 57 Co in Rh matrix. The velocity scale was calibrated relative to α-Fe foil, and the spectrum was collected over 18 h. Based on conventional Mössbauer spectroscopic analyses, we determined that Fe in the synthesized glass was mainly present in the Fe 2+ state, and the Fe 3+ content of the glass was below the detection limit, consistent with the conditions during synthesis. A multicomponent silicate glass with basaltic composition (M-glass; Table 1 ) was synthesized from a mixture of oxides at 1 GPa and 1,400 °C in a piston-cylinder press using a graphite capsule. The composition and homogeneity of the final glasses were confirmed by electron probe microanalysis and by observation using a polarized optical microscope. Optical absorption measurements Optical absorption measurements were conducted on E-glass up to 65 GPa and M-glass up to 80 GPa in the near-infrared to visible spectrum at the Geophysical Laboratory, Carnegie Institution of Washington. A doubly polished, optically clear glass sample with 15 μm thickness was loaded into a symmetric-type diamond anvil cell (DAC) with 300 μm culets using a neon pressure medium ( Fig. 1 ). Several ruby spheres were placed around the sample, and pressure was determined using the pressure-dependent energy shift of the R 1 ruby fluorescence line. The details of the methods and error analysis applied in the present optical absorption measurements are described elsewhere [11] , [12] , [32] . Visible spectra were acquired using the 300 grooves per millimetre grating with a 0.5-m single-stage grating monochromator. A combined deuterium and halogen lamp was used as the light source for optical absorption measurements and was directed to a focused spot diameter of ~20 μm at the sample inside the DAC. Unpolarized near-infrared spectra were obtained with a Varian Resolution Pro 670-IR spectrometer. At each pressure, absorption spectra through the sample and the reference spectrum through diamond and neon pressure medium were obtained for the flat-field correction. The experimental error has a maximum value of ~0.05 absorbance units owing to the non-reproducibility in sample position and vignetting of the probing beam [32] . Scattering losses in the sample and in the medium are very small for the materials used. A double pinhole geometry was used in our measurements that effectively blocks all spurious light. The angle of incidence of light in air is <16°. Inside the sample, this angle is even smaller, thereby allowing description of the incident light with a nearly normal propagation direction. The maximum angle of light in the sample is less than 16° per refractive index n . With n ~2 this would equal an angle of 8°, which changes the path length by ~1%, which is negligible [32] . The reflection losses ( A R ) derived from our measurements were calculated using the method previously proposed [13] . The net result of this approximation is found to be A R =0.010(1) in absorbance units. The sum of experimental uncertainties can contribute up to ~10% error in calculated conductivity values. Synchrotron Mössbauer spectroscopic measurements In situ high-pressure synchrotron Mössbauer spectroscopic measurements were undertaken on E-glass at the BL11XU beamline of a third-generation synchrotron radiation facility of SPring-8 (ref. 26 ). Using energy-domain synchrotron Mössbauer spectroscopy and focusing X-ray optics, 57 Fe Mössbauer transmission spectra of samples of E-glass were collected in a DAC from 20 to 85 GPa without a pressure medium. In this experimental setup, a liquid nitrogen-cooled Si(111) double-crystal monochromator was used to handle the high heat load of undulator radiation, and a σ-polarized beam in 57 Fe was produced by a nested high-resolution monochromator consisting of asymmetric Si(511) and asymmetric Si(975) channel-cut crystals. A small-size probe beam was produced by a bent elliptical multilayer X-ray focusing mirror that was coated with 50 layers of W (13 Å)/Si (39.5 Å) on a high-quality quartz SiO 2 base. Then, the incident X-rays were reflected at a Bragg peak angle and were horizontally focused at the sample position. The ultrahigh monochromatic X-rays with energy width ~15 neV were produced by a nuclear analyser crystal using the electrically forbidden (333) pure nuclear Bragg reflection from a 57 FeBO 3 single crystal near the Néel temperature in an external magnetic field of 150 Gauss. The nuclear Bragg-diffracted X-rays were detected by a NaI scintillation detector. The Mössbauer spectrum was measured by counting the intensity of single-line nuclear Bragg reflection as a function of velocity. How to cite this article : Murakami, M. et al . High-pressure radiative conductivity of dense silicate glasses with potential implications for dark magmas. Nat. Commun. 5:5428 doi: 10.1038/ncomms6428 (2014).